Cryptic prophages help bacteria cope with adverse environments Phages are the most abundant entity in the biosphere and outnumber bacteria by a factor of 10. Phage DNA may also constitute 20% of bacterial genomes; however, its role is ill defined. Here, we explore the impact of cryptic prophages on cell physiology by precisely deleting all nine prophage elements (166 kbp) using Escherichia coli . We find that cryptic prophages contribute significantly to resistance to sub-lethal concentrations of quinolone and β-lactam antibiotics primarily through proteins that inhibit cell division (for example, KilR of rac and DicB of Qin). Moreover, the prophages are beneficial for withstanding osmotic, oxidative and acid stresses, for increasing growth, and for influencing biofilm formation. Prophage CPS-53 proteins YfdK, YfdO and YfdS enhanced resistance to oxidative stress, prophages e14, CPS-53 and CP4-57 increased resistance to acid, and e14 and rac proteins increased early biofilm formation. Therefore, cryptic prophages provide multiple benefits to the host for surviving adverse environmental conditions. The term prophage was coined in 1952 by André Lwoff, who along with François Jacob and Jacques Monod, discovered that phages use lysogeny (incorporation into the chromosome) as a means to replicate, and who believed that lysogeny is a window into our understanding of the relationship between bacteria and phages [1] . Because of their prevalence, acquisition of prophages contributes most to the horizontal gene transfer, as phage-like elements have been identified in almost all sequenced pathogenic and non-pathogenic bacterial genomes, and can constitute up to 20% of the DNA [2] even though bacteria have compact genomes. Although it has been reasoned for decades that metabolically inert prophage DNA would cause a selective disadvantage to the host [3] , the role of much of this prophage material remains largely unknown. Prophages may become trapped in the chromosome of the host due to various genome rearrangements and gradual decay [4] and become inactive in terms of cell lysis, phage particle production and plaque formation; these prophage elements are referred to as cryptic prophages (we use active prophage here to indicate prophage capable of forming plaques). The well-studied Escherichia coli K-12 has gained 1,600 kbp of novel DNA (18%) since its divergence from Salmonella sp. 100 million years ago [5] and contains nine cryptic prophage elements, which comprise 3.6% of its genome. Clearly prophage rac is a DNA fossil as it was acquired over 4.5 million years ago [6] . Most examples indicating a role of prophages in cell physiology involve active prophage; these include the Bor protein of phage lambda, which increases the survival of E. coli by providing resistance to serum-mediated killing [7] . Along with lambda, active Mu, P1 and P2 prophages also increase growth under glucose-limited growing conditions [3] , [8] , and we have shown that cryptic prophage CP4-57 increases cell growth in several media [9] . In addition, prophage-encoded virulence factors make important contributions to pathogenesis including those of Corynebacterium diphtheriae (diphtheria), Clostridium botulinum (botulism) and E. coli O157:H7 (Shiga-like toxin) [10] . Active prophages such as Gifsy-2 can also give the Salmonella host a competitive advantage by killing competitors and by providing immunity [11] . In these cases, the reproductive success of the lysogenic bacterium carrying these new genes translates directly into an evolutionary success for the prophage resident in the chromosome. With the emergence of global systems biology tools such as DNA microarrays, cryptic prophage genes have gradually gained attention, as part of host physiology, especially under conditions where the cells are stressed such as those that exist in biofilms [12] . Our goal here was to begin to understand the evolutionary importance of cryptic prophage elements by exploring the function of prophage genes on cell physiology. To this end, we created a single E. coli strain, Δ9, that lacks all nine cryptic prophages (CP4-6, DLP12, e14, rac, Qin, CP4-44, CPS-53, CPZ-55 and CP4-57); each prophage was removed precisely using a method that leaves one attachment site and mimics natural excision. Two systems biology tools, phenotype and DNA microarrays, were then used to identify the altered phenotypes and to elucidate the important prophage genes responsible for the changes in the phenotypes. Strikingly, we determined that the poorly studied cryptic prophage genes increased growth, provided protection for quinolone and β-lactam antibiotics, increased resistance to osmotic, oxidative and acid stress, as well as influenced biofilm formation. Therefore, these cryptic prophage genes have a profound, beneficial impact on cell physiology. Prophages increase cell growth To assess the overall effect of harbouring nine cryptic prophages ( Fig. 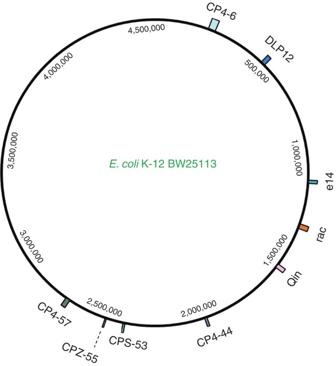Figure 1: Size and position of nine cryptic prophages in theE. coliK-12 BW25113 genome. Map of theE. coliK-12 BW25113 genome demonstrating the cyptic prophages deleted in this study. 1 ) on E. coli host physiology, growth of the Δ9 strain ( Table 1 ) was tested in nutrient-rich medium at 37 °C (to mimic conditions that E. coli should encounter in the gastrointestinal tract) and in nutrient-poor medium at 30 °C (to mimic the cooler temperatures likely to be experienced by E. coli outside the human host). The maximum specific growth rates for Δ9 were decreased slightly in both media (1.36±0.01 versus 1.46±0.02 h −1 in rich medium and 0.25±0.02 versus 0.28±0.01 h −1 in minimal medium for Δ9 and the wild-type strain, respectively); however, the prophage-deleted cells had decreased yields on these substrates ( Fig. 2a,b ). 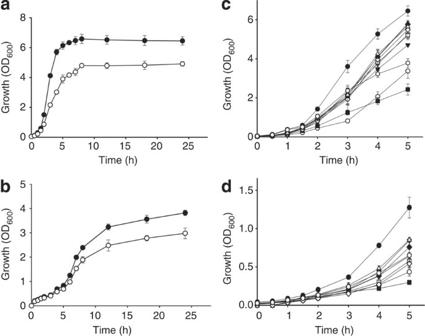Figure 2: Cryptic prophage genes influence cell growth. Growth in LB at 37 °C (a) and M9C at 30 °C (b) for Δ9 (open circle) and the wild-type strain (filled circle). Growth of the nine individual prophage deletion strains (CP4-6, open diamond; DLP12, filled diamond; e14, open hexagon; rac, inverted open triangle; Qin, filled triangle; CPS-53, inverted filled triangle; CP4-44, open square; CPZ-55, open triangle and CP4-57, filled square), Δ9 (open circle) and the wild-type strain (filled circle) in LB at 37 °C (c) and M9C lactate at 37 °C (d). Error bars indicate s.d. values (n=3). In addition, growth of each of the nine individual prophage-deletion strains ( Table 2 ) was tested. Among the nine strains, growth in both media was reduced the most on removing CP4-57 ( Fig. 2c,d ). Hence, prophages confer the ability to grow more rapidly and to obtain higher yields on nutrients. Figure 1: Size and position of nine cryptic prophages in the E. coli K-12 BW25113 genome. Map of the E. coli K-12 BW25113 genome demonstrating the cyptic prophages deleted in this study. Full size image Table 1 The genes in each cryptic prophage and the method used to remove each of the nine prophages from E. coli K-12. Full size table Figure 2: Cryptic prophage genes influence cell growth. Growth in LB at 37 °C ( a ) and M9C at 30 °C ( b ) for Δ9 (open circle) and the wild-type strain (filled circle). Growth of the nine individual prophage deletion strains (CP4-6, open diamond; DLP12, filled diamond; e14, open hexagon; rac, inverted open triangle; Qin, filled triangle; CPS-53, inverted filled triangle; CP4-44, open square; CPZ-55, open triangle and CP4-57, filled square), Δ9 (open circle) and the wild-type strain (filled circle) in LB at 37 °C ( c ) and M9C lactate at 37 °C ( d ). Error bars indicate s.d. values ( n =3). Full size image Table 2 E. coli K-12 bacterial strains and plasmids used in this study. Full size table Prophages increase resistance to quinolone antibiotics To examine the impact of deleting the nine cryptic prophages on specific aspects of E. coli physiology, we used phenotype microarrays (PMs) so that 1,240 different metabolic conditions could be rapidly assayed in a high-throughput manner [13] ; this method both amplifies and quantifies the differences in metabolism of the strains. Using plates PM 11–13, six quinolone antibiotics (four shown in Fig. 3a and six in Supplementary Table S1 ) dramatically inhibited the growth of Δ9 at concentrations that are 1/2 of the minimum inhibitory concentration (MIC) for the wild-type strain. These include first generation oxolinic acid and nalidixic acid, second-generation enoxacin, lomefloxacin and ofloxacin, and the related novobiocin agent. Quinolones are broad-spectrum antibacterial agents that are becoming increasingly popular and account for 18% of the antibacterial market (2006) [14] . 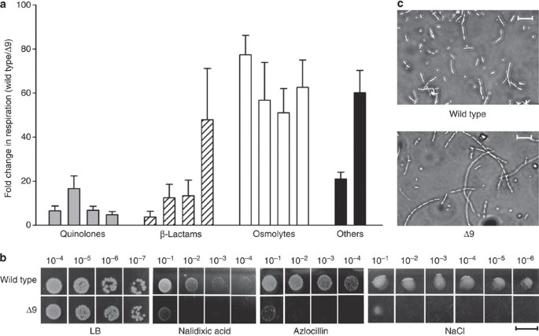Figure 3: Cryptic prophage genes influence stress-related phenotypes. (a) Summary of the PM results for the wild-type strain versus Δ9. The fold changes indicate the relative difference in the average slope in the growth curves multiplied by the area under the curves, which is indicative of cell respiration. From left to right, with the MIC indicated for the wild-type strain in parenthesis, quinolones include nalidixic acid (4 μg ml−1), oxolinic acid (0.9 μg ml−1), ofloxacin (0.048 μg ml−1) and novobiocin (132 μg ml−1); β-lactams include nafcillin (320 μg ml−1), azlocillin (17.6 μg ml−1), cephalothin (5.12 μg ml−1) and moxalactam (0.27 μg ml−1); osmolytes include 5% NaCl, 6% NaCl, 6% KCl and 2% sodium formate; and the other stresses include thallium acetate and potassium tellurite. All chemicals shown here were significantly repressed for Δ9 versus wild-type strain (P<0.05 using a pairedt-test). Error bars indicate s.e.m. (n=3). (b) Efficiency of colony formation for Δ9 and the wild-type strain with sublethal concentrations of nalidixic acid (2 μg ml−1) and azlocillin (5 μg ml−1) as well as with 6% NaCl. Powers of 10 indicate the amount of dilution. Scale bar represents 10 mm. (c) Cell morphology for Δ9 and wild-type strain after treating with 2 μg ml−1nalidixic acid for 2 h. Scale bar represents 10 μm. Figure 3: Cryptic prophage genes influence stress-related phenotypes. ( a ) Summary of the PM results for the wild-type strain versus Δ9. The fold changes indicate the relative difference in the average slope in the growth curves multiplied by the area under the curves, which is indicative of cell respiration. From left to right, with the MIC indicated for the wild-type strain in parenthesis, quinolones include nalidixic acid (4 μg ml −1 ), oxolinic acid (0.9 μg ml −1 ), ofloxacin (0.048 μg ml −1 ) and novobiocin (132 μg ml −1 ); β-lactams include nafcillin (320 μg ml −1 ), azlocillin (17.6 μg ml −1 ), cephalothin (5.12 μg ml −1 ) and moxalactam (0.27 μg ml −1 ); osmolytes include 5% NaCl, 6% NaCl, 6% KCl and 2% sodium formate; and the other stresses include thallium acetate and potassium tellurite. All chemicals shown here were significantly repressed for Δ9 versus wild-type strain ( P <0.05 using a paired t -test). Error bars indicate s.e.m. ( n =3). ( b ) Efficiency of colony formation for Δ9 and the wild-type strain with sublethal concentrations of nalidixic acid (2 μg ml −1 ) and azlocillin (5 μg ml −1 ) as well as with 6% NaCl. Powers of 10 indicate the amount of dilution. Scale bar represents 10 mm. ( c ) Cell morphology for Δ9 and wild-type strain after treating with 2 μg ml −1 nalidixic acid for 2 h. Scale bar represents 10 μm. Full size image To confirm the results from the PM assays, the MIC 99 of nalidixic acid, defined as the lowest drug concentration that inhibits growth by 99% [15] , was measured, and a 2.1-fold decrease in the MIC 99 of Δ9 was found (3.9 μg ml −1 ) compared with the wild-type strain (8.0 μg ml −1 ). Note that MIC values are based on turbidity so they do not discriminate between bactericidal or bacteriostatic action [16] . Therefore, to further assess the bactericidal action of quinolone antibiotics, cell viability of the wild-type strain and Δ9 were also tested with 2 μg ml −1 nalidixic acid. Critically, the viability of Δ9 was repressed 379-fold for 2 μg ml −1 nalidixic acid ( Fig. 3b ); hence, the relatively small change in MIC is not representative of the large effect on cell viability caused by the prophage. A similar large change in viability was seen previously with a relatively small change in MIC for nalidixic acid and a defect in chromosome partitioning [17] . In Gram-negative bacteria, quinolone targets DNA gyrase and triggers an SOS response (global response to DNA damage) at sub-lethal concentrations [18] . Induction of the SOS response in E. coli causes inhibition of cell division via FtsZ [19] . Thus, the cell morphology of exponentially growing wild-type and Δ9 cells treated with 2 μg ml −1 nalidixic acid for 2 h was examined, and it was found that Δ9 cells are more elongated than the wild-type strain ( Fig. 3c ). Hence, the increased filamentous growth in Δ9 confirms inhibition of cell division when cells encounter DNA gyrase inhibitors [20] and β-lactams [21] . Although cells grow as elongated filaments when septation is inhibited, these filamented cells will eventually lyse [22] , [23] and decrease the number of viable cells as seen in Figure 3b . Without the addition of nalidixic acid, both wild-type and Δ9 cells have normal morphology. To explore the impact of the individual prophage on resistance to nalidixic acid (2 μg ml −1 ), strains with a single prophage deleted were tested. We determined that prophages CP4-6 and rac were primarily responsible for the enhanced resistance to nalidixic acid (33- and 41-fold, respectively; Fig. 4a ). 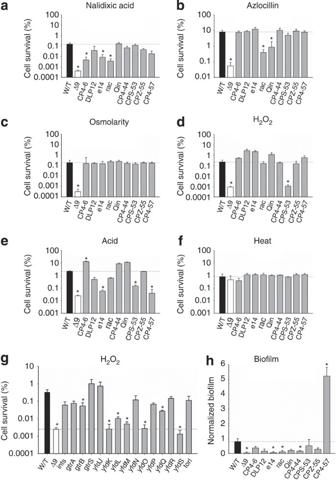Figure 4: Individual prophages affect cell viability with stress and biofilm formation. Survival for the nine single-prophage deletion strains (marked with each prophage name) and the multiple prophage-deletion strain (Δ9) after challenging with (a) nalidixic acid (2 μg ml−1for 12 h), (b) azlocillin (4 μg ml−1for 12 h), (c) osmotic stress (6% NaCl for 12 h), (d) oxidative stress (30 mM H2O2for 15 min), (e) acid stress (pH 2.5 for 30 min) and (f) heat stress (65 °C for 10 min). (g) Survival for the 15 single-gene deletion strains of CPS-53 (marked with each gene deletion) and the multiple prophage-deletion strain (Δ9) after challenging with oxidative stress (30 mM H2O2for 15 min). (h) Normalized biofilm formation in 96-well polystyrene plates in M9C medium after 8 h at 30 °C. Error bars indicate s.d. values (n=4). Significant changes are marked with an asterisk forP<0.05. Figure 4: Individual prophages affect cell viability with stress and biofilm formation. Survival for the nine single-prophage deletion strains (marked with each prophage name) and the multiple prophage-deletion strain (Δ9) after challenging with ( a ) nalidixic acid (2 μg ml −1 for 12 h), ( b ) azlocillin (4 μg ml −1 for 12 h), ( c ) osmotic stress (6% NaCl for 12 h), ( d ) oxidative stress (30 mM H 2 O 2 for 15 min), ( e ) acid stress (pH 2.5 for 30 min) and ( f ) heat stress (65 °C for 10 min). ( g ) Survival for the 15 single-gene deletion strains of CPS-53 (marked with each gene deletion) and the multiple prophage-deletion strain (Δ9) after challenging with oxidative stress (30 mM H 2 O 2 for 15 min). ( h ) Normalized biofilm formation in 96-well polystyrene plates in M9C medium after 8 h at 30 °C. Error bars indicate s.d. values ( n =4). Significant changes are marked with an asterisk for P <0.05. Full size image Prophages increase resistance to β-lactam antibiotics The lethality of β-lactam antibiotics stems from their interaction with transmembrane penicillin-binding proteins and the consequent disruption of cell wall integrity for fast-growing strains [24] . β-Lactam antibiotics, when used at sublethal concentrations, also induce an SOS response [25] . The PM assay showed that removing all nine prophages decreased resistance to 11 β-lactam antibiotics, including the most common penicillins and cephalosporins (four shown in Fig. 3a and nine in Supplementary Table S1 ), which accounted for 17 and 27% of sales in the antibacterial market in 2006, respectively [14] . To confirm the PM results, the MIC 99 of azlocillin was also measured, and a 3.9-fold reduction in the MIC 99 of Δ9 was found (4.8 μg ml −1 ) compared with the wild-type strain (18.6 μg ml −1 ). The cell viability of the wild-type strain and Δ9 were tested using 5 μg ml −1 azlocillin and 20 μg ml −1 ampicillin, and the growth of Δ9 was repressed by 146-fold ( Fig. 3b ) and 52-fold, respectively. Therefore, similar to its interaction with quinolones, the prophage-deleted strain is more sensitive to β-lactam antibiotics. To identify which cryptic prophages are primarily responsible for the decreased resistance of Δ9 to azlocillin, each of the single prophage-deletion strains was tested. Deletion of prophages of rac and Qin caused lower resistance to 4 μg ml −1 azlocillin (20- and 9-fold, respectively; Fig. 4b ). Induction of prophage genes by antibiotics To identify specific genes within the individual prophages that are affected by the quinolone and β-lactam antibiotics, a whole-transcriptome study was performed in response to subinhibitory concentrations of nalidixic acid (2 μg ml −1 ) and azlocillin (10 μg ml −1 ). For nalidixic acid, 17 prophage genes were induced >2.5-fold out of a total of 95 induced genes, and for azlocillin, 43 prophage genes were induced >2.5-fold out of a total of 168 induced genes ( Supplementary Table S2 ). Putative cell division inhibitor genes were induced by both nalidixic acid and azlocillin including kilR from rac, dicB , dicC and dicF from Qin, and ymfL and ymfM from e14, Lambdoid kil genes can inhibit cell division to maintain synchrony with the host in its lysogenic state [26] , and lambdoid prophage rac has a functional kilR gene that seems to cause cell division arrest [27] . DicB from Qin can rapidly cease cell division by targeting FtsZ when it is induced under stress [28] . In addition, lambdoid prophage e14 has a functional division inhibition gene encoded by ymfL or ymfM (ref. [29] ). To further study the role of these genes in response of Δ9 to azlocillin (5 μg ml −1 ), cell viability on deleting kilR , ymfL , ymfM , dicB and dicC were tested. Compared with the wild-type strain, deletion of dicB greatly reduced cell viability after exposure to azlocillin (82-fold), whereas deletion of dicC had no effect. Deletion of rac gene kilR also significantly reduced cell viability (fivefold), and reduced the colony size as seen for Δ9 ( Fig. 3b ). Deletion of ymfL and ymfM did not significantly reduce cell viability to azlocillin. Similarly for nalidixic acid (2 μg ml −1 ), deletion of dicB and kilR significantly reduced cell viability 4- and 35-fold, whereas the deletion of other five genes had little effect. Hence, DicB and KilR are responsible for much of the enhanced resistance to azlocillin and nalidixic acid, and these results are expected given that the rac and Qin prophages were found to be most important when the single prophage deletion strains were evaluated for their effect on antibiotic stress ( Fig. 4b ). Consistent with the whole-transcriptome study, quantitative real-time reverse-transcription PCR (qRT–PCR) confirmed that kilR and dicB were both induced in cells treated with nalidixic acid (21±1- and 33±2-fold, respectively) and with azlocillin (18±1- and 35±2-fold, respectively). As for Δ9 ( Fig. 3c ), increased cell elongation was also observed for the kilR and dicB mutants 2 h after the addition of sublethal concentrations of nalidixic acid (2 μg ml −1 ) and azlocillin (5 μg ml −1 ). Therefore, induction of these single genes from two cryptic prophages that encode division inhibitors increases survival against quinolone and β-lactams antibiotics and affects cell division. Prophages increase resistance to environmental stresses Phenotype microarray PM9 is designed for testing osmotic and ion sensitivity; using this plate, we found that when exposed to a high-salt environment (for example, 6% NaCl and 6% KCl), the metabolism of Δ9 was totally inhibited, whereas the wild-type strain adapted to this stress and grew well ( Fig. 3a,b , Supplementary Table S1 ). These results were corroborated using shake flasks in that osmotic stress (6% NaCl for 12 h) reduced the cell survival of Δ9 by 787-fold ( Fig. 4c ). Similarly, we found that the growth of Δ9 was inhibited with the addition of potassium tellurite ( Fig. 3a ) whose toxicity in E. coli involves oxidative stress [30] . On the basis of this result, we tested the resistance of Δ9 to oxidative stress (30 mM H 2 O 2 for 15 min), acid stress (pH 2.5 for 30 min), and heat (65 °C for 10 min). Removing of all nine prophages significantly decreased resistance to oxidative stress (245-fold; Fig. 4d ) and acid stress (90-fold; Fig. 4e ); however, there was no difference in the ability of Δ9 to withstand heat stress ( Fig. 4f ). Therefore, the presence of prophages dramatically improves the ability of the cell to withstand osmotic, oxidative and acid stress. To probe the impact of the individual prophage on stress resistance, strains with a single prophage deleted were tested for sensitivity to acid, heat, osmotic stress and oxidative stress. For acid stress ( Fig. 4e ), removing e14, CPS-53 and CP4-57 significantly decreased resistance by 38-, 15- and 56-fold, respectively. For osmotic and heat stress ( Fig. 4c,f ), there was little effect of deleting each individual prophage. For oxidative stress ( Fig. 4d ), the absence of prophage CPS-53 alone almost accounted for all of the sensitivity of Δ9. To determine which specific proteins of prophage CPS-53 are responsible for the increased resistance to oxidative stress, we tested all of the CPS-53 genes for their effect on oxidative stress resistance and found that deletion of yfdK , yfdO and yfdS reduced viability similar to Δ9 ( Fig. 4g ). The function of the proteins encoded by the CPS-53 genes is unknown. Hence, we identified specific proteins related to the change in the oxidative stress phenotype seen on deleting the nine prophages. As RpoS is the master regulator of the stationary stress response [31] and positively regulates genes necessary for the oxidative stress response such as katE [32] , which encodes catalase, and oxyR , which encodes a regulatory protein sensor for oxidative stress [32] , we tested the impact of deleting CPS-53 on the transcription of rpoS , katE and oxyR . qRT–PCR showed that transcription of rpoS , oxyR and katE was repressed (4±1-, 3±1- and 3±1-fold, respectively) in ΔCPS-53 compared with the wild-type strain when treated with 2 mM H 2 O 2 . Therefore, these results link prophage CPS-53 to RpoS and serve to explain why cells without CPS-53 have reduced viability when challenged with H 2 O 2 . Prophages increase biofilm formation Biofilms are the preferred lifestyle of bacteria [33] ; therefore, we tested biofilm formation after deleting the nine cryptic prophages. In minimal medium, biofilm formation was almost completely abolished for Δ9 compared with the wild-type strain ( Fig. 4h ). Hence, prophages enhance the ability of E. coli to form biofilms. To probe the impact of the individual prophage on biofilm formation, strains with a single prophage deleted were tested for biofilm formation in minimal medium. Deletion of eight prophages independently decreased early biofilm formation by 3- to 11-fold, but deletion of prophage CP4-57 increased early biofilm formation by 6±2-fold; this increase in biofilm formation on deleting CP4-57 explains the reduction in growth of planktonic cells ( Fig. 2c,d ). Removing prophages e14, rac and CP4-44 had the greatest impact on reducing biofilm formation ( Fig. 4h ). The reduction in the early biofilm formation of Δ9 is likely due to the reduced cell aggregation compared with the wild-type strain ( Supplementary Fig. S1 ), as aggregation is directly related to biofilm formation. As the deletion of e14 and rac affected biofilm formation to the largest extent, we examined each gene of these two prophages (47 genes) for their impact on biofilm formation and determined deletion of intE and ymfD of e14 and intR , stfR , ydaF , ydaS and ydaW of rac reduced early biofilm formation to the level seen with Δ9. These results are consistent with the results that the removal of intA encoding CP4-57 integrase and intD encoding DLP12 integrase affect early biofilm formation [9] . In addition, we found that ymfD and stfR are induced in mature biofilms in a temporal microarray study [12] . Prophage excision To test the stability and excision proficiency of each of the nine prophages, the fraction of cells that undergoes excision was quantified by quantitative PCR in a total of |10 10 cells. The size and the position of each prophage is shown in Figure 1 and Table 1 . In exponentially growing cells, seven of the nine prophages excised ( Fig. 5 ). Prophage e14 had the highest excision rate (1–5 per 10,000 cells), and CP4-6 and rac had an excision frequency of tenfold lower (1–27 per 100,000 cells). DLP12, CPS-53, CPZ-55 and CP4-57 also excised, but with very low frequencies (<1 per 100,000 cells). In contrast, excision of Qin and CP4-44 was not detected. This is expected because the integrase for Qin ( intQ ) is inactive [34] , and CP4-44 lacks an integrase [35] . These results indicate these prophages are stable under exponential growth. 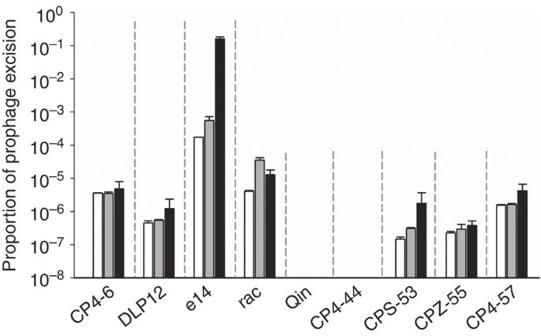Figure 5: Prophage excised at different frequencies. Proportion of wild-type cells that have the indicated prophage excised without mitomycin C (open bar), with the addition of 1 μg ml−1of mitomycin C (grey bar) and 10 μg ml−1of mitomycin C (black bar). Mitomycin C was added to exponential-phase cells (turbidity |1.0) in LB medium at 37 °C for 4 h. Error bars indicate s.d. values (n=3). Figure 5: Prophage excised at different frequencies. Proportion of wild-type cells that have the indicated prophage excised without mitomycin C (open bar), with the addition of 1 μg ml −1 of mitomycin C (grey bar) and 10 μg ml −1 of mitomycin C (black bar). Mitomycin C was added to exponential-phase cells (turbidity |1.0) in LB medium at 37 °C for 4 h. Error bars indicate s.d. values ( n =3). Full size image To test excision under adverse conditions, mitomycin C was used; this antibiotic induces the DNA repair (SOS) response in bacteria and converts lysogenic phages to the lytic form [34] . e14 was the only inducible prophage on mitomycin C treatment, and its excision rate increased up to 356-fold, which led to 13% of the cells losing e14 ( Fig. 5 ). Similar results were found with an oxidative stress challenge. These results again indicate these prophages are stable except for e14. The nine different prophages in E. coli K-12 have been captured at different stages of evolution, which is reflected by their different excision rates ( Fig. 5 ). It seems that both Qin and CP4-44 have been enslaved by the host and trapped in the chromosome in a permanent state of lysogeny. Except for e14, the other eight prophages have lost the ability to excise on SOS response challenge, which is known to trigger active prophages to excise from the host [36] . Therefore, the prophages studied here are phage fossils, as they have lost the ability to excise and form phage particles, and now suffer the same fate as the host. However, rather than serving the prophages, their genes now serve the host. The beneficial impacts of the cryptic prophage genes on cell physiology include enhanced growth in rich and minimal media ( Fig. 2 ), enhanced phosphorus and nitrogen utilization, and most importantly, the cryptic prophage genes increase the host's response to general environmental stress (for example, oxidative, acidic and osmotic stress) and to antibiotics (quinolones and β-lactams) ( Figs 3 and 4 ). Not surprisingly, these prophage genes are non-essential, and thus, dispensable under common culturing conditions, based on cell growth and cell respiration in the majority of the PM assays. Using plates PM 1–8 which assay nutrient utilization, only 16 out of 760 (2%) conditions inhibited the respiration of Δ9 >threefold, whereas using plates PM 9–13, which assay sensitivity to stress, 73 out of 480 (15%) conditions inhibited respiration of Δ9 >threefold. These results agree well with those of even larger scale genome deletions (up to 15% of the genome) in E. coli K-12 MG1655, which were performed in an effort to engineer a reduced E. coli genome [37] , [38] ; these deletions did not compromise essential host physiological functions under standard culturing conditions. PM assays 1–4, which test for growth differences in carbon, nitrogen, phosphorous and sulphur sources, showed MDS12 had reduced growth for 15 conditions [38] . In contrast, we found that Δ9 had reduced growth for five conditions and had increased growth for four conditions. The major difference between mutant MDS12 (376,183 bp removed) [37] , [38] and Δ9 (166,481 bp removed) is that we constructed a nine prophage-deletion strain with precise removal of each prophage in a manner which mimics natural excision leaving one attachment site for each prophage, whereas MDS12, which was constructed for different aims, has deleted not only prophage DNA but also neighbouring regions [37] . The precise deletions here allowed us to study the impact of the prophages without the effects of flanking host gene regions. For example, cryptic prophages Qin, CP4-44 and CPZ-55 integrate into non-regulatory intergenic regions or pseudogenes so the host is not affected. Furthermore, three of the cryptic prophages (CP4-6, DLP12 and CPS-53) integrate into tRNA genes ( CP4-6 , DLP12 and CPS-53 ) and reconstitute a functional tRNA gene after integration; hence, their removal leaves the same functional tRNA, and the host was not altered in this regard when we deleted these prophages. Prophages e14 and rac integrate into structural genes that encode isocitrate dehydrogenase and a tRNA 2-thiocytidine biosynthesis protein, respectively, by inserting a homologous sequence on integration to maintain protein activity. Natural excision of e14 and rac restores both genes to their native versions [39] . CP4-57 integrates into the tmRNA gene ssrA and its excision leaves a transcriptionally active ssrA with a one base pair change [9] ; we checked the importance of SsrA by deleting ssrA and found this had no impact on the cell's response to nalidixic acid and osmotic stress. Therefore, we have constructed the first strain devoid solely of phage elements larger than a single gene to study their impact on cell physiology. Although we cannot rule out that our deletion of the prophage genes may have altered some suppressor interactions with host genes, it seems clear, based on the specific genes we identified, that some of the phage-encoded genes are functional and are responsible for the phenotypes seen here. Different from well-studied Shiga-like toxin encoding E. coli in which toxin release relies on prophage induction [40] , with the exception of e14, the influence of these genes on E. coli K-12 cell physiology does not seem to rely on excision ( Fig. 5 ); hence, there are cryptic prophage genes that confer a benefit to the host in a manner different from their expression as part of a phage that was once capable of causing cell lysis. Instead, individual genes are expressed in cryptic prophage even though the prophage on the whole is no longer active; this concept is related to the genes of active prophage that are transcribed independently of plaque formation and that were theorized to provide benefits during lysogeny [10] . Our work extends this concept and identifies several proteins in the cryptic prophages that benefit the host and do so in terms of stress resistance. Other key proteins that may be related directly to the phenotypes explored here include four toxin/antitoxin (TA) systems that are located in the prophages including the well-studied RelEB [41] (Qin) and three recently identified TA pairs YpjF-YfjZ (CP4-57), YkfI-YafW (CP4-6) and YeeV-YeeU (CP4-44) [42] . We have found the MqsR/MqsA TA system of E. coli aids in the survival against some antibiotics due to persister cell formation [43] . In addition, 24 cryptic prophage genes have been linked to persistence, including the relE toxin gene of Qin and the yeeV toxin gene of CP4-44 [44] . Furthermore, we have linked TA systems to biofilm formation [45] . Hence, TA systems may be important here for the biofilm and general stress response phenotypes. In addition, as TA genes from bacterial prophages are actively expressed in the human gastrointestinal tract, TA systems may have a dynamic role in different ecosystems [46] . Indubitably, other uncharacterized genes in these cryptic prophages might also contribute to the stress response of the host, and there are probably intricate regulation mechanisms that need to be investigated. The most striking result of this study is that cryptic phage fossils help the host cope with stress. Here, we show that cryptic prophages, instead of being passive genetic cargo of the bacterial genome, help the cell respond to various stresses as active loci. Evolutionary forces promote bacterial growth in many environmental niches, so survival under difficult conditions is crucial. Thus, it is not surprising that bacteria adapt to their environment; for example, they frequently become resistant to antimicrobial agents [47] . Our results suggest that phages and their resulting lysogeny may serve as an important means for bacteria to gain greater fitness. It has been theorized that the introduction of novel genes by phage can confer beneficial phenotypes that allow the exploitation of competitive environments [4] , and the results here support this hypothesis. Specifically, we show that the emergence of resistance to both antibiotics as well as to environmental stress arises in some cases from the acquisition of phage DNA. This suggests that inhibiting key proteins encoded by prophages may be a novel means to combat antibiotic resistance. In effect, the cell uses the tools it obtained from its former enemy, phage, to cope with new environments. Bacterial growth and plasmids The isogenic E. coli BW25113 K-12 strains and plasmids used in this study are listed in Table 2 . For deleting and overexpressing genes, we used the Keio collection [48] and the ASKA library [49] . All experiments were conducted at 37 °C, except for growth in M9C and for biofilm formation, which were conducted at 30 °C (to create more stress). Luria–Bertani (LB) medium [50] , M9 minimal medium with 0.2% casamino acids (M9C) [51] and M9C with 0.1% lactate (M9C lactate) were used as indicated. Kanamycin (50 μg ml −1 ) was used for preculturing isogenic knockout mutants, chloramphenicol (30 μg ml −1 ) was used for maintaining pCA24N-based plasmids and ampicillin (100 μg ml −1 ) was used to maintain plasmids pKD46 and pCP20. Construction of single prophage deletion mutants Prophage deletion strains ΔCP4-57, ΔCPS-53, Δe14 and Δrac were obtained by overexpressing alpA, which encodes AlpA that causes excision [9] , torI (encodes excisionase) [52] , intE (encodes integrase) [29] and engineered hns that induces rac prophage excision [53] , respectively, from pCA24N-derived plasmids [49] ( Table 2 ). This process is equivalent to natural excision and leads to a host genome devoid of both prophages and phage-like circles. To facilitate the screening of the loss of each of these prophages from the host genome, a Keio strain [48] that has kanamycin resistance marker inside each prophage was used; colonies were screened for the loss of kanamycin resistance after induction of integrase or excisionase by 1 mM IPTG for 4–8 h. Complete removal of each prophage was confirmed by PCR followed by DNA sequencing using primers flanking each prophage ( Supplementary Table S3 ); this sequencing confirmed an attachment site was retained in the host after each prophage excision, which confirmed no additional nucleotide sequences were deleted in the host. To delete (individually) the remaining five prophages, a second approach was used in which we expanded the use of the one-step inactivation method that was originally used for single-gene deletions [54] . After one-step inactivation using primers flanking the prophage ( Supplementary Table S3 ), the whole DLP12 prophage (21,302 bp) was replaced with a kanamycin resistance cassette (1.5 kbp) from plasmid pKD4. The primers were designed to keep only one attachment site (5′ site) in the E. coli host genome after each knockout, which mimics natural excision. After deleting each cryptic prophage, the kanamycin gene was removed by using the Flp recombinase sites that flank the kanamycin resistance gene; this leaves 85 bp of pKD4 next to the remaining prophage attachment site. In an analogous manner, prophages Qin (20,458 bp), CP4-6 (34,308 bp), CP4-44 (13,152 bp) and CPZ-55 (6,763 bp) were individually removed from the wild-type strain (primer pairs shown in Supplementary Table S3 ). The replacement of prophage with the kanamycin resistance marker and its removal were confirmed by PCR followed by DNA sequencing primers flanking the prophage sequences ( Supplementary Table S3 ). Removal of all nine prophages To form a strain that is devoid of all nine cryptic prophages but that does not contain any other mutations, termed Δ9, we started with the single deletion prophage strain Δrac, then by overexpressing torI and alpA in succession, we obtained Δrac ΔCPS-53 ΔCP4-57 (Δ3) that lacks the entire rac, CPS-53 and CP4-57 prophage regions. P1 transduction [55] was used next to transfer rapidly the ΔDLP12 Km R mutation to Δ3 to obtain strain Δ4. The kanamycin resistance cassette from the newly constructed multiple deletion strain Δ4 was removed by plasmid pCP20, and this strain was used as a recipient for P1 transduction to transfer ΔQin Km R . Prophage e14 was removed by overproducing IntE. CPZ-55, CP4-6 and CP4-44 were sequentially removed by P1 transduction, resulting in strains Δ7, Δ8 and, finally, strain Δ9, which lacks all nine prophages. The final full deletion strain was checked by PCR to confirm the removal of 166 kbp of prophage and prophage-like elements (3.6% of the genome) from E. coli K-12 to create the first E. coli strain solely devoid of prophages ( Table 1 ). As expected, all 203 genes of the nine cryptic prophages in Δ9 had an expression level of zero in an E. coli GeneChip Genome 2.0 microarray (Affymetrix, P/N 4059655). Crystal violet biofilm assay Biofilm formation was assayed in 96-well polystyrene plates (Corning Costar) with crystal violet staining [56] . To remove growth effects, biofilm formation was normalized by dividing total biofilm by bacterial growth for each strain. Growth and stress assays Growth was determined using turbidity measurements at 600 nm with LB, M9C and M9C lactate. MIC 99 values for nalidixic acid and azlocillin were determined with an initial inoculum of 5×10 5 cells per ml using the broth dilution method [16] with the modifications of using shaking (250 r.p.m.) and LB medium. For testing the efficiency of colony formation (cell viability) under different conditions, exponential growing cells (turbidity |0.5) were diluted and cultured on LB plates with sublethal concentrations of antibiotics (nalidixic acid, ampicillin and azlocillin) as well as 6% NaCl (LB plates were used as a control). For the stress assays, H 2 O 2 , heat, acid and NaCl were added to cells growing in the early exponential stage (turbidity |0.5), and cell viability was determined by serial dilutions on LB agar plates. Cell morphology of the wild-type, Δ9, kilR and dicB strains was examined 2 h after the addition of 2 μg ml −1 nalidixic acid and 5 μg ml −1 azlocillin to exponentially growing cells (turbidity |0.5) using a Zeiss Axiovert 200 microscope (Zeiss). Phenotype microarrays Δ9 and the wild-type strain were assayed for differences in metabolism using microplates PM1 to PM13 from Biolog. PM1 and PM2 contain 190 alternative C-sources, PM3, 6, 7 and 8 contain 380 alternative N-sources, PM4 and PM5 contain phosphorus, sulphur and other nutrient-supplying pathways, PM9 contains tests for osmotic and ion effects, PM10 contains tests for pH effects, and PM11, 12 and 13 contain chemicals that provide information on stress and repair pathways that are active in cells [57] . PM technology uses the irreversible reduction of tetrazolium violet to formazan as a reporter of active metabolism [57] ; the purple colour generated is recorded every 15 min and provides quantitative and kinetic information about the response of the cells. All procedures were performed as indicated by the manufacturer, and the data were analysed using OminoLog software. For each well, the product of the area and the average slope of the time course data were used to score cell respiration [58] . RNA isolation and whole-transcriptome studies RNA was isolated from BW25113 incubated with 2 μg ml −1 nalidixic acid, 10 μg ml −1 azlocillin or no antibiotic after 90 min (antibiotics added when the turbidity was ~0.8). As the antibiotic concentrations used were below the MIC values, growth (as indicated by the turbidity) was comparable with and without antibiotics. Total RNA was isolated using a bead beater (Biospec) and was converted into cDNAs through a reverse transcription reaction with poly(A) RNA controls [59] . The cDNAs were then digested with DNase I (Amersham Biosciences) to produce 50- to 200-bp fragments, the fragmented cDNAs were labelled with biotin, and the labelled cDNAs were hybridized at 45 °C for 16 h to the E. coli GeneChip Genome 2.0 array (Affymetrix, P/N 511302) [59] 59. The gene expression data are accessible through GEO accession number GSE23359. Quantitative real-time PCR (qPCR) To determine the prophage excision rate, the number of chromosomes that are devoid of each prophage was quantified using primers flanking each prophage ( Supplementary Table S3 ), which only give PCR products when the prophage is removed because of the size of the prophage ( Table 1 ). The relative amount of each target gene was determined using reference gene purA . Total DNA (50–200 ng) was isolated using an UltraClean Microbial DNA Isolation Kit (Mo Bio Laboratories) and used as the template for the qPCR reaction using the SuperScript III Platinum SYBR Green One-Step qRT–PCR Kit (Invitrogen). The reaction and analysis was conducted using the StepOne Real-Time PCR System (Applied Biosystems). Quantitative real-time reverse-transcription PCR Different from the qPCR described above, which determined the relative concentrations of specific DNA fragments, qRT-PCR was used to quantify relative RNA concentrations using 50 ng as a template and included a complementary DNA synthesis step from RNA before the denaturation step. Primers for qRT-PCR for kilR , dicB , rpoS , oxyR and katE are listed in Supplementary Table S3 . The housekeeping gene rrsG (16S rRNA gene) was used to normalize the gene expression data. How to cite this article: Wang, X. et al . Cryptic prophages help bacteria cope with adverse environments. Nat. Commun. 1:147 doi: 10.1038/ncomms1146 (2010).